Identification of evolutionarily conserved regulators of muscle mitochondrial network organization Mitochondrial networks provide coordinated energy distribution throughout muscle cells. However, pathways specifying mitochondrial networks are incompletely understood and it is unclear how they might affect contractile fiber-type. Here, we show that natural energetic demands placed on Drosophila melanogaster muscles yield native cell-types among which contractile and mitochondrial network-types are regulated differentially. Proteomic analyses of indirect flight, jump, and leg muscles, together with muscles misexpressing known fiber-type specification factor salm , identified transcription factors H15 and cut as potential mitochondrial network regulators. We demonstrate H15 operates downstream of salm regulating flight muscle contractile and mitochondrial network-type. Conversely, H15 regulates mitochondrial network configuration but not contractile type in jump and leg muscles. Further, we find that cut regulates salm expression in flight muscles and mitochondrial network configuration in leg muscles. These data indicate cell type-specific regulation of muscle mitochondrial network organization through evolutionarily conserved transcription factors cut , salm , and H15 . Proper mitochondrial network formation and maintenance are crucial for cellular energy distribution, cell signaling, and movement of ions, metabolites, mtDNA, and proteins [1] , [2] , [3] , [4] , [5] , [6] . Mitochondrial network structure is highly variable across cell types due to differences in the amount of cellular volume allotted to mitochondria, the size and shape of individual mitochondria, and the configuration or location of mitochondria within the cell, with each of these structural parameters influencing the relative efficiency of interaction and communication among mitochondria and other cellular structures [7] , [8] , [9] , [10] . While regulators of cellular mitochondrial volume (e.g., PGC-1, ERR, and PPAR isoforms) and individual mitochondrial size (e.g., Drp1, Mfn1/2, and Fis1) have been widely identified and studied across cell types [11] , [12] , [13] , [14] , [15] , [16] , [17] , [18] , [19] , [20] , [21] , [22] , [23] , how mitochondrial network configuration is determined as part of the cellular design process is less well understood [24] , [25] , [26] . Mature striated muscles form relatively stable mitochondrial networks [27] comprised of many physically and electrically connected mitochondria [5] , [28] , [29] , and muscle mitochondrial networks display differences in mitochondrial content, size, and configuration depending on the energetic and contractile force requirements of a given muscle cell type [5] , [28] , [30] , [31] , [32] . In mammalian systems, muscle type is commonly classified by both contractile (i.e., fast- or slow-twitch) and metabolic (i.e., glycolytic or oxidative) types [33] , [34] with contractile type generally defined by myosin isoform composition or myofibrillar ATPase activity [35] , [36] , [37] and metabolic type often inferred based on mitochondrial content or enzyme activity [35] , [38] , [39] , [40] . Due to the intimate structural and functional relationships between the contractile [41] and mitochondrial networks, it is not surprising that many of the well-known factors involved in muscle fiber type specification can regulate the design of both the contractile and metabolic machineries within the muscle cell [42] , [43] , [44] , [45] . Conversely, there are also many examples of alterations in muscle metabolism, mitochondrial content, and mitochondrial size without affecting contractile fiber type [11] , [15] , [46] , [47] , [48] , [49] , [50] , [51] , [52] , [53] , [54] , [55] , [56] demonstrating that muscle metabolism and mitochondrial structure can be regulated independently of contractile type. In order to identify regulators of muscle mitochondrial network configuration, particularly with respect to their impact on contractile type, our first aim was to establish a model system allowing for rapid screening of potential regulatory genes or proteins. Unfortunately, commonly used muscle cell culture models (e.g., myoblasts or myotubes) feature underdeveloped contractile networks permitting frequent mitochondrial movement around the cell which makes these systems ineffective for assessment of regulators of the configuration of the relatively static mitochondrial networks observed in adult muscles [27] . As a result, we turned to the genetically tractable fruit fly, Drosophila melanogaster , where mitochondrial structure and metabolism have been widely studied in the adult indirect flight muscles [15] , [46] , [47] , [54] , [55] , [57] , [58] , [59] , [60] . Though contractile characteristics have been assessed across many different adult Drosophila muscles [61] , [62] , [63] , [64] , much less information is available regarding metabolism or mitochondria in adult Drosophila muscles beyond the flight muscles [50] , [65] . Indeed, in contrast to mammalian systems, muscle cell type in Drosophila muscles has been largely defined by contractile (i.e., fibrillar or tubular) or electromechanical (i.e., synchronous or asynchronous) properties rather than metabolic characteristics [63] , [66] , [67] , [68] , [69] . Though the indirect flight muscles are the largest and most well-studied muscles in Drosophila , the fibrillar (i.e., comprised of individual myofibrils) and asynchronous (i.e., one calcium cycle results in tens of muscle contractions) nature of these muscles are unlike any known mammalian muscle. Conversely, the majority of Drosophila muscles are tubular [70] (i.e., form cross-striated myofibrillar networks [32] ) and synchronous (i.e., one calcium cycle per contraction) more similar to mammalian skeletal muscles. Despite being classified as the same contractile type, tubular muscles can have different contractile characteristics (e.g., mechanical force/power [61] , [62] , [63] , [64] and sarcomere [71] or myofibrillar network [32] structure) consistent with the variable functions of each specific Drosophila muscle. We hypothesized that, like mammals, the wide variety of contractile demands faced across Drosophila tubular muscles would also necessitate cells of varying oxidative or glycolytic natures, and in turn, muscles with different mitochondrial network configurations. Thus, we aimed to identify Drosophila muscles with differing mitochondrial network structures and use this multi-muscle system to screen for genetic regulators of mitochondrial network configuration. Moreover, we sought to determine whether any newly identified genes regulate mitochondrial network configuration in coordination with contractile type (i.e., muscle converts between fibrillar and tubular types) or independently of contractile type (i.e., muscle remains fibrillar or tubular). Here, we take advantage of the natural energetic and contractile differences [61] , [63] among muscle types within the genetically tractable fruit fly, Drosophila melanogaster , together with the known Drosophila muscle type specification factor, spalt major ( salm ) [50] , [67] to identify evolutionarily conserved regulators of muscle mitochondrial network organization. By performing a proteomic screen on muscles with five different combinations of contractile type, mitochondrial network type, and Salm expression level, we identified 142 proteins associated with muscle fiber type. Further, we demonstrate that H15 is a regulatory transcription factor downstream from salm which can independently regulate contractile type or mitochondrial network configuration in a muscle type-specific manner. Moreover, we show that transcription factor cut operates upstream of salm and can also independently regulate mitochondrial network configuration in a muscle type-specific manner. Finally, we demonstrate that the specification of mitochondrial network configuration in muscles can be regulated separately from cellular mitochondrial volume and individual mitochondrial volume. Our findings suggest that evolutionarily conserved transcription factors including cut , salm , and H15 regulate mitochondrial network configuration in muscle cells through a specification process which can operate independently of contractile type, mitochondrial content, and mitochondrial size. Wild-type mitochondrial network and contractile types To monitor mitochondrial and contractile network morphology in the different muscle types in Drosophila , we used the genetically encoded mitochondrial matrix GFP [72] with the UAS-Gal4 system [47] together with F-actin staining (Phalloidin). The indirect flight muscles (dorsal longitudinal muscles (DLMs)) in wild-type adult flies showed the characteristic fibrillar contractile phenotype of many individual myofibrils [67] , [73] together with many thick, elongated mitochondria interspersed in parallel to the myofibrils (Fig. 1a–d,u ) (Supplementary Movie 1 ). Flight muscles also had relatively low sarcoplasmic reticulum (SR) content as assessed with genetically encoded KDEL-RFP (Fig. 1e, v and Fig. S 1a–c ). On the other hand, the jump (tergal depressor of the trochanter (TDT)) muscles exhibited closely aligned myofibrils representative of their tubular contractile phenotype combined with fewer thin, elongated mitochondria also arranged in parallel to the axis of muscle contraction (Fig. 1f–i, u ) (Supplementary Movie 2 ) and high SR content (Fig. 1j, v and Fig. S 1d–f ). In the leg muscles (coxa of the forelegs), we consistently observed different phenotypes in three spatially distinct regions we termed Fibers I, II, and III (Fig. 1k–q ). All three leg regions displayed tubular myofibrils (Fig. 1m, o, q , and Fig. S 2 ). However, Fiber I had primarily parallel mitochondrial networks (Fig. 1l,u ) (Supplementary Movie 3 ) and lower mitochondrial content (Fig. 1t ) compared to the more grid-like networks in Fibers II and III (Fig. 1m, n, p, u ) (Supplementary Movies 4 and 5 ). All three leg regions had higher SR content than the flight muscles (Fig. 1v and Fig. S 1g–r ). The grid-like nature of the mitochondrial networks in the tubular leg muscles (Fiber II and III, Fig. 1r ), the parallel mitochondrial networks in the fibrillar flight (Fig. 1d ) and tubular jump muscles (Fig. 1i ), and the relative differences in SR content were confirmed by focused ion beam scanning electron microscopy (FIB-SEM, Fig. 1e, j, s ). These data from wild-type fly muscles show that parallel mitochondrial networks can occur together with either fibrillar (flight) or tubular (jump) contractile types and that tubular muscles can have either parallel (jump/leg Fiber I) or grid-like mitochondrial networks (leg Fiber II/III) (Fig. S 3 ), demonstrating that contractile type and metabolic phenotypes can be regulated independently in Drosophila muscles. Fig. 1: Mitochondrial network organization in adult Drosophila muscles. a , b , c Fibrillar flight muscles (IFMs) stained for F - actin and mitochondria expressing mito-gfp driven by DMef2-Gal4 showing parallel aligned mitochondria that are large, tube-like, and packed between myofibrils (Scale Bars: 5 μm). d , e Representative 3D rendering of electron microscopic images of mitochondrial arrangement (yellow) and ER (magenta) in flight muscles. f , g , h Tubular jump muscles show mitochondria that are thin and elongated arranged in parallel mitochondrial networks (Scale Bars: 5 μm). i , j Representative 3D rendering of mitochondrial networks (yellow) and ER (magenta) in jump muscles. k In walking (leg) muscles, DMef2-Gal4 driven mito-gfp shows both parallel and grid-like mitochondrial networks (marked with dashed line, scale bar: 20 μm). l , m Tubular leg muscle Fiber I showing primarily parallel mitochondrial networks. n , o Tubular leg muscle Fiber II showing a grid-like mitochondrial network. p , q Tubular leg muscle Fiber III showing grid-like mitochondria. (Scale Bars: 5 μm for all). r , s Representative 3D rendering of mitochondrial network organization (yellow) and ER (magenta) in leg muscles. t Mitochondrial volume as a percent of total muscle volume (Flight muscles (IFM) ( UAS-mito-gfp;Dmef2-Gal4 ), n = 5 animals; Jump muscles (TDT) ( UAS-mito-gfp;Dmef2-Gal4), n = 5 animals; Leg Fiber I, n = 7 animals; Leg Fiber II, n = 9 animals; Leg Fiber III, n = 5 animals). u Quantification of mitochondrial network orientation. Dotted line represents parallel equal to perpendicular (IFM, n = 11 animals; Jump muscles (TDT), n = 12 animals; Leg Fiber I, n = 10 animals; Leg Fiber II, n = 9 animals; Leg Fiber III, n = 6 animals). v Endoplasmic reticulum (ER) volume as a percent of total muscle volume (IFM, n = 5 animals; Jump muscles (TDT), n = 5 animals; Leg Fiber I, n = 3 animals; Leg Fiber II, n = 4 animals; Leg Fiber III, n = 5 animals). Each point represents value for each animal dataset. Bars represent mean ± SD. Significance determined as p < 0.05 from one way ANOVA with Tukey’s (*, p ≤ 0.05; **, p ≤ 0.01; ***, p ≤ 0.001; ****, p ≤ 0.0001; ns, non-significant). Full size image Regulators of mitochondrial networks in fly muscles Mitochondrial dynamics proteins have been implicated in mitochondrial network formation across many cell types [20] , [22] , [74] , [75] , [76] , [77] . Thus, we initially attempted to alter mitochondrial network configuration by knocking down mitochondrial dynamics proteins which promote mitochondrial fusion (Marf, mfn1/2 ortholog), mitochondrial fission (Drp1 and Fis1), and mitochondrial motility (Miro) in a muscle-specific manner (using Mef2-Gal4 ). Loss of Marf is sufficient to induce smaller, more circular mitochondria (Fig. S 4c, m, n ), lower mitochondrial volume (Fig. S 4o ), and the complete loss of flight and climbing ability (Fig. S 5a, b ). However, Marf KD did not change the orientation of mitochondrial networks in either the flight or Fiber II leg muscles (Fig. S 5d, k, l ). Reductions in fission proteins Drp1 and Fis1 to levels sufficient to cause larger, more elongated mitochondria (Fig. S 4e, g, m, n ) affected neither mitochondrial network configuration (Fig. S 4f, h, o ) nor flight or climbing ability (Fig. S 5a, b ). Finally, loss of Miro also resulted in smaller, more circular mitochondria (Fig. S 4i, m, n ) and a complete lack of flight and climbing ability (Fig. S 5a, b ), but did not alter mitochondrial network configuration (Fig. S 4j, k, l ). These results indicate that individual mitochondrial size can be up or down-regulated without altering mitochondrial network configuration in muscle cells. Next, we examined the role of zinc finger transcription factor salm in the regulation of muscle-specific mitochondrial network organization, by performing salm misexpression in Drosophila muscles. Salm is a known regulator of fibrillar muscle fate in Drosophila [67] , and recently was reported to be involved in specifying mitochondrial location in flight muscles [50] . As shown previously [78] , salm was highly expressed in the wild-type flight muscles (Fig. S 6a–d ), while lower levels of salm expression were observed in wild type jump muscles (Fig. S 6e–h ) and expression was undetectable in wild type leg muscles (Fig. S 6i–l ). Muscle-specific RNAi-mediated salm knockdown using Mef2-Gal4 (Fig. S 6m–p ) resulted in flightless flies with a reduced jumping ability (Fig. S 5a, c ) and conversion of the flight muscle contractile apparatus to tubular muscle and the mitochondrial networks to grid-like (Fig. 2a–h,o ). It is important to note that salm KD mediated conversion of muscle type occurs whether one ( UAS-salm RNAi , Figs. S 6 , 7 ) or two ( UAS-salm RNAi::UAS-mito-GFP , Fig. 2f–h ) UAS are present. Additionally, the fiber transformation in salm KD flight muscles was accompanied by an increase in ER content to the level of the wild type tubular muscles (Fig. S 7j–l ). On the other hand, salm KD had no effect on the contractile type or mitochondrial morphology in the jump or leg muscles (Fig. S 7d, e, h , and Fig. S 8a–d ). These results are consistent with salm as a critical specification factor between flight and leg muscle phenotypes. Fig. 2: salm regulates conversion of muscle fiber contractile type and mitochondrial network orientation. a Adult wild-type flight muscles (fibrillar) stained for F-actin (phTRITC). b salm KD muscle fiber stained for muscles showing tubular muscle type (Scale Bars: 100 μm). c , d , e Wildtype flight muscles show elongated, parallel mitochondria (mito-gfp) between myofibers (phTRITC). f , g , h The knockdown of salm (UAS-salm RNAi;UAS-mito-gfp;mef2) in flight muscles results in fiber conversion to tubular muscle type and mitochondria to a grid-like network. (i) Wild type leg muscles show tubular muscle type in the coxa. Inset shows a cross-section of leg muscles displaying well-aligned fibers. j , k Wildtype leg muscles show parallel mitochondria (mito-mcherry) aligned next to myofibrils (phTRITC). l salm OE converts muscle fibers to fibrillar in nature. Inset, well-defined fibrillar fibers in cross-section of leg muscles. m , n salm OE leg muscles have parallel mitochondrial networks (mito-mcherry) along the myofibrils (phTRITC) (Scale Bars: 5 μm for all). o Quantification of mitochondrial network orientation. Dotted line represents parallel equal to perpendicular. mito-gfp;mito-mcherry;mef2-Gal4 used as Wildtype, WT. (WT-IFM, n = 9 animals; salm -KD IFM, n = 7 animals; WT-Leg Fiber I, n = 6 animals; salm -OE Leg Fiber I, n = 8 animals). Each point represents value for each animal dataset. Bars represent mean ± SD. Significance determined as p < 0.05 from one way ANOVA with Tukey’s (*, p ≤ 0.05; **, p ≤ 0.01; ***, p ≤ 0.001; ****, p ≤ 0.0001; ns, non-significant). Full size image To investigate the impact of increased salm expression on mitochondrial network organization, we overexpressed (OE) salm in Drosophila muscles (Fig. S 6q–t ). salm OE in muscles resulted in pupal lethality and escapers showed dysfunctional walking behavior (100%, Fig. S 5b ). Importantly, salm OE transformed the tubular leg myofibrils to more fibrillar-like myofibrils similar to those in flight muscles (Fig. 2i, l ). However, following salm OE, the mitochondrial networks in the transformed leg muscles remained similar to those in wild type tubular walking muscle fibers as there was no significant difference in the ratio of parallel to perpendicular mitochondria compared to wild type leg muscles (Fig. 2i–o ). In the salm OE studies, we used Tom20-mcherry instead of mito-GFP as the genetically encoded mitochondrial reporter because UAS-mito-GFP , as well as Tub-Gal80ts and UAS-salm used for salm OE, are located on the same chromosome. However, no differences in the mitochondrial network configuration were observed across muscle types between mito-GFP and Tom20-mcherry reporters (Fig. S 9 ), suggesting that neither the choice of mitochondrial marker nor the use of a second UAS influenced our network orientation results. Additionally, salm OE had no apparent effect on the parallel mitochondrial networks in the jump muscle or flight muscle (Fig. S 8e, g ). Overall, these results demonstrate that salm is a critical factor in determining mitochondrial network organization in flight muscles and in determining contractile type in both flight and leg muscles, but salm does not appear to play a key role in jump muscle contractile or metabolic specification. Proteomic screen for factors associated with fiber type To identify additional potential regulators of muscle fiber type specification, we performed a high-throughput, TMT-based [79] proteomic screen on the three wild-type muscles (flight, jump, leg) (Fig. 1 ) together with the two muscles which underwent fiber type conversion with salm misexpression ( salm KD flight, salm OE leg) (Fig. 2 ). A total of 3869 proteins were quantified for each sample (Supplemental Data 1 ). While the overall protein abundance profile of each sample was similar (Fig. S 10a ), principal component and heat map clustering analyses indicated strong reproducibility and clear distinctions among the five muscle types assessed (Fig. S 10b, c ). To characterize the differences among muscle types, differentially expressed proteins (Fig. S 11 ) were run through a gene enrichment analysis using g:Profiler [80] and primarily identified myofibrillar and mitochondrial processes, consistent with our phenotypic image analyses above (Fig. S 12 ). 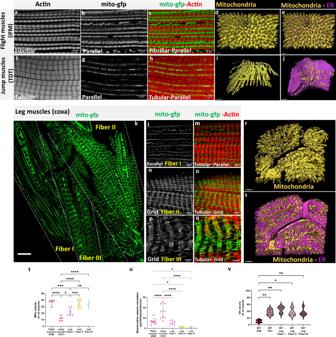Fig. 1: Mitochondrial network organization in adult Drosophila muscles. a,b,cFibrillar flight muscles (IFMs) stained for F - actin and mitochondria expressing mito-gfp driven byDMef2-Gal4showing parallel aligned mitochondria that are large, tube-like, and packed between myofibrils (Scale Bars: 5 μm).d,eRepresentative 3D rendering of electron microscopic images of mitochondrial arrangement (yellow) and ER (magenta) in flight muscles.f,g,hTubular jump muscles show mitochondria that are thin and elongated arranged in parallel mitochondrial networks (Scale Bars: 5 μm).i,jRepresentative 3D rendering of mitochondrial networks (yellow) and ER (magenta) in jump muscles.kIn walking (leg) muscles,DMef2-Gal4driven mito-gfp shows both parallel and grid-like mitochondrial networks (marked with dashed line, scale bar: 20 μm).l,mTubular leg muscle Fiber I showing primarily parallel mitochondrial networks.n,oTubular leg muscle Fiber II showing a grid-like mitochondrial network.p,qTubular leg muscle Fiber III showing grid-like mitochondria. (Scale Bars: 5 μm for all).r,sRepresentative 3D rendering of mitochondrial network organization (yellow) and ER (magenta) in leg muscles.tMitochondrial volume as a percent of total muscle volume (Flight muscles (IFM) (UAS-mito-gfp;Dmef2-Gal4),n= 5 animals; Jump muscles (TDT) (UAS-mito-gfp;Dmef2-Gal4), n= 5 animals; Leg Fiber I,n= 7 animals; Leg Fiber II,n= 9 animals; Leg Fiber III,n= 5 animals).uQuantification of mitochondrial network orientation. Dotted line represents parallel equal to perpendicular (IFM,n= 11 animals; Jump muscles (TDT),n=12animals; Leg Fiber I,n= 10 animals; Leg Fiber II,n= 9 animals; Leg Fiber III,n= 6 animals).vEndoplasmic reticulum (ER) volume as a percent of total muscle volume (IFM,n=5animals; Jump muscles (TDT),n=5animals; Leg Fiber I,n= 3 animals; Leg Fiber II,n= 4 animals; Leg Fiber III,n=5animals). Each point represents value for each animal dataset. Bars represent mean ± SD. Significance determined asp< 0.05 from one way ANOVA with Tukey’s (*,p≤ 0.05; **,p≤ 0.01; ***,p≤ 0.001; ****,p≤ 0.0001; ns, non-significant). To identify regulators specific for each muscle mitochondrial network configuration and/or contractile type, we rationalized that by assessing protein expression in muscles each with varying combinations of mitochondrial network configuration (parallel or grid-like), contractile type (fibrillar or tubular), and salm expression (Supplementary Table 1 ), we could make multiple comparisons of differentially expressed proteins associated with a given phenotype and identify proteins which were consistently associated across all comparisons. For example, we hypothesized that proteins positively associated with fibrillar muscle fate (Fibrillar+) would be higher in wild type flight muscles compared with wild type leg (558 proteins), wild type jump (1326 proteins), or salm KD flight muscles (597 proteins) and in salm OE leg muscles compared to wild type leg muscles (1387 proteins) (Fig. 3a ). Of all the proteins identified by each individual comparison, 25 proteins were consistently found across all four Fibrillar+ comparisons (Fig. 3a ). To determine proteins negatively associated with fibrillar muscle fate (Fibrillar-), the inverse analysis was performed by identifying proteins that were lower in the wild type flight muscles compared to wild type leg (2450 proteins), wild type jump (771 proteins), or salm KD flight muscles (1674 proteins) and in salm OE leg muscles compared to wild type leg muscles (590 proteins) yielding 2 proteins that were consistent across all Fibrillar- comparisons (Fig. 3b ). Similar analyses identified 6 Tubular+ proteins (Fig. 3c ), 7 Tubular- proteins (Figs. 3 d), 3 Parallel+ proteins (Fig. 3e ), 23 Parallel- proteins (Fig. 3f ), 565 Grid+ proteins (Fig. 3g ), 9 Grid- proteins (Figs. 3 h), 1 salm+ protein (Fig. 3i ), and 50 salm- proteins (Fig. 3j ). The relatively large number of Grid+ proteins is due in part to having only three rather than four or five comparisons groups like for the other phenotypes (Fig. 3 ). As a result, we further filtered the Grid+ proteins down to 16 using the microarray data from Schonbauer et al [67] ., which reported transcripts with higher expression levels in two muscles shown here to have grid-like mitochondrial networks, the wild type leg and salm KD flight muscles, relative to wild type flight muscles. Thus, in total, we identified 142 proteins whose expression levels consistently correlated with at least one fiber type specification phenotype (Supplemental Data 2 ). Fig. 3: Identification of potential regulatory factors for contractile and mitochondrial network type in Drosophila muscle. a Venn diagram displaying the individual muscle group comparisons and their overlap for proteins positively associated with fibrillar muscles. b Venn diagram displaying the individual muscle group comparisons and their overlap for proteins negatively associated with fibrillar muscles. c , d Venn diagram for tubular positively and negatively associated proteins, respectively. e , f Venn diagram for positively and negatively associated proteins, respectively, with parallel mitochondrial networks. g , h Venn diagram for positively and negatively associated proteins, respectively, with grid-like mitochondrial networks. i , j Venn diagram for salm positively and negatively associated proteins, respectively. Full size image H15 regulates muscle fiber type downstream of salm Of the 51 salm -associated proteins, there was only one Salm+ protein, H15, which met the thresholds of our screen. H15 is a T-box transcription factor, orthologous to the vertebrate proteins, Tbx20 and Tbx15 . Importantly, Tbx15 has been suggested to regulate glycolytic fiber-type specification in a whole-body knockout model in the mouse [81] , though how Tbx15 interacts with other transcription factors to specify muscle cell fate remains unclear. Based on the positive association with salm expression, we hypothesized that H15 would regulate fiber type specification downstream of salm in Drosophila muscles and provide further support for the evolutionarily conserved nature of the salm -associated regulation of mitochondrial network configuration identified in Drosophila muscle. To assess the impact of H15 on mitochondrial network organization and muscle contractile specification in muscles, we first performed muscle-specific H15 KD using Mef2-Gal4 during Drosophila muscle development. We initially tested two different H15 KD lines (V28415, V106875) and found that the V28415 H15 KD line led to viable flightless adults (Fig. S 5a ) whereas the V106875 H15 KD line resulted in weak flight. Thus, we chose the stronger phenotype (V28415) for all further H15 KD analyses. H15 KD was confirmed by immunofluorescence (Fig. S 18a–h, z ) and resulted in contractile type switching of the flight muscle fibers from fibrillar to tubular (Fig. 4a, d ) (Fig. S 13e–h ). Further quantitative qPCR analysis showed significant decrease in fibrillar sarcomeric transcript expression, Flightin (fln), troponin C (Tpnc4), and Actin88F (Fig. S 13i ). Moreover, mitochondrial content was significantly reduced in the flight muscles following H15 KD (15.59 ± 1.13% of muscle volume) when compared to the wild-type flight muscles (38.88 ± 0.9%, Fig. S 14a ), and the mitochondrial networks remained organized parallel to the axis of contraction similar to wild type flight and jump muscles (Fig. 4a–f ). Indeed, there was no significant difference in the ratio of parallel to perpendicular mitochondria between H15 KD and wild-type flight muscles (Fig. 4s ). Thus, in contrast to salm KD, H15 KD induced a jump muscle phenotype (tubular/parallel) rather than a leg muscle phenotype (tubular/grid) in the flight muscles indicating that mitochondrial network configuration can be regulated independently from contractile type in the flight muscle. Fig. 4: H15 independently regulates the conversion of muscle contractile type and mitochondrial network configuration in Drosophila muscles. a , b , c Fibrillar flight muscles (IFMs) stained for F-actin (phTRITC) and mitochondria (mito-GFP) showing parallel aligned mitochondria between myofibrils. d H15 KD shows fibrillar muscles switched to tubular muscle type. e , f H15 KD muscles show parallel mitochondria along muscle fibers. g , h , i Tubular jump muscles show parallel mitochondria (thin and elongated). j H15 KD in jump muscles shows tubular fibers (phTRITC). k , l Upon H15 KD, tubular jump muscles show a change in mitochondrial networks to more grid-like (Scale Bars: 5 μm for all). m Wildtype coxa leg muscle Fiber I showing parallel mitochondrial networks. n Wildtype leg muscle Fiber II and o Fiber III showing grid-like mitochondrial networks. p H15 KD leg muscle Fiber I showing conversion to a grid-like mitochondrial network. q , r H15 KD leg muscle fibers II and III show grid-like structures similar to their wild type counterparts (Scale Bars: 5 μm for all). s Quantification of mitochondrial network orientation. Dotted line represents parallel equal to perpendicular. mito-gfp;mito-mcherry;mef2-Gal4 used as wildtype, WT; indirect flight muscles, IFM; Jump muscles, TDT. (WT-IFM, n = 9 animals; H15 KD-IFM, n = 6 animals; WT-TDT, n = 8 animals; H15 KD-TDT, n = 8 animals). t Quantification of mitochondrial network orientation in leg (walking) Fibers. (WT-leg Fibers I, n = 5 animals; H15 KD-IFM, n = 7 animals; WT-leg Fiber II, n = 9 animals; H15 KD-Leg Fiber II, n = 5 animals; WT-Leg Fiber III, n = 6 animals, H15 KD-Leg Fiber III, n = 5 animals). Each point represents value for each dataset. Bars represent mean ± SD. Significance determined as p < 0.05 from one way ANOVA with Tukey’s (*, p ≤ 0.05; **, p ≤ 0.01; ***, p ≤ 0.001; ****, p ≤ 0.0001; ns, non-significant). Full size image In the jump muscles, H15 KD did not appear to affect the tubular nature of the myofibrils (Fig. 4g, j ). However, H15 KD converted the parallel mitochondrial networks to a more grid-like arrangement (Fig. 4g–l ) (Supplementary Movie 6 ) as evident in the decrease in the ratio of parallel to perpendicular mitochondria in H15 KD jump muscles compared to wild-type jump muscles (Fig. 4s ) (Supplementary Movie 2 ). Thus, loss of H15 in the jump muscles resulted in a phenotype similar to the wild-type leg muscles (Fiber II, III tubular/grid) and was accompanied by a reduction in jumping ability (Fig. S 5c ). These results suggest that H15 regulates mitochondrial network configuration but not contractile type in the jump muscles. However, it should be noted that while H15 KD does not alter the tubular contractile type of the jump muscles, muscle-specific loss of H15 has recently been shown to increase sarcomere branching frequency [32] and myosin filament curvature [71] above the level of the wild-type jump muscles and closer to the levels of the wild type leg muscles. Those results are consistent with the interpretation here that H15 KD in the jump muscle results in a leg muscle-like phenotype based on the tubular contractile type and grid-like mitochondrial networks. In the leg muscles following H15 KD, the contractile structure was clearly tubular in all three fiber regions (Fig. S 15l, o, r ). However, knockdown of H15 transformed the parallel mitochondrial networks of Fiber I in the leg to a grid-like organization (Fig. 4m, p ) (Supplementary Movie 7 ), as confirmed by the decrease in the ratio of parallel to perpendicular mitochondria compared to the wild type leg muscle Fiber I (Fig. 4t ). Conversely, H15 KD did not affect the grid-like mitochondrial networks of Fiber II and Fiber III (Fig. 4q, r, t ), which remained similar to those in the wild type leg muscles (Fig. 4n, o, t ). These data further suggest that H15 regulation of mitochondrial network organization occurs in a cell-type-specific manner and can operate independently of contractile type specification. 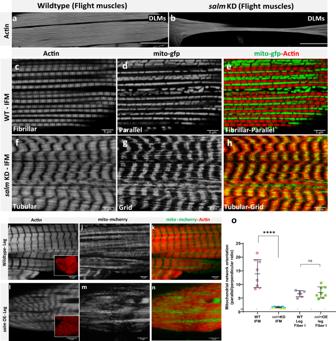Fig. 2:salmregulates conversion of muscle fiber contractile type and mitochondrial network orientation. aAdult wild-type flight muscles (fibrillar) stained for F-actin (phTRITC).bsalmKD muscle fiber stained for muscles showing tubular muscle type (Scale Bars: 100 μm).c,d,eWildtype flight muscles show elongated, parallel mitochondria (mito-gfp) between myofibers (phTRITC).f,g,hThe knockdown ofsalm (UAS-salm RNAi;UAS-mito-gfp;mef2)in flight muscles results in fiber conversion to tubular muscle type and mitochondria to a grid-like network. (i) Wild type leg muscles show tubular muscle type in the coxa. Inset shows a cross-section of leg muscles displaying well-aligned fibers.j,kWildtype leg muscles show parallel mitochondria (mito-mcherry) aligned next to myofibrils (phTRITC).lsalmOE converts muscle fibers to fibrillar in nature. Inset, well-defined fibrillar fibers in cross-section of leg muscles.m,nsalmOE leg muscles have parallel mitochondrial networks (mito-mcherry) along the myofibrils (phTRITC) (Scale Bars: 5 μm for all).oQuantification of mitochondrial network orientation. Dotted line represents parallel equal to perpendicular.mito-gfp;mito-mcherry;mef2-Gal4used as Wildtype, WT. (WT-IFM,n= 9 animals;salm-KD IFM,n=7animals; WT-Leg Fiber I,n=6animals;salm-OE Leg Fiber I,n=8animals). Each point represents value for each animal dataset. Bars represent mean ± SD. Significance determined asp< 0.05 from one way ANOVA with Tukey’s (*,p≤ 0.05; **,p≤ 0.01; ***,p≤ 0.001; ****,p≤ 0.0001; ns, non-significant). To test whether the flight muscle contractile phenotype was specifically due to H15 down-regulation rather than off-target effects, individual Mef2 -Gal4 driven knockdowns of 16 genes that are off-targets of the H15 RNAi line (VDRC 28415) were evaluated based on a previous flight muscle genetic screen [82] and our own imaging of eight different knockdowns (Supplemental Table 2 ). Downregulation of these off-targets did not cause a tubular conversion of the flight muscles (Fig. S 16 ), though loss of CG31374 ( sals ) led to partial lethality with eclosing flies unable to fly likely related to the apparent shortening and thinning of the sarcomeres as reported previously [83] . In addition, we also assessed the role of mid , a paralog of H15 , in mitochondrial network organization and muscle contractile specification in muscles and found that mid KD did not cause conversion of myofibrillar or mitochondrial networks in flight, jump and leg fiber I muscles (Fig. S 17 ). These results suggest that the muscle type conversions observed in the H15 KD flies are mediated specifically by H15 rather than off-target or paralogous genes. To test our hypothesis that H15 operates downstream of salm in Drosophila muscle, we first assessed Salm and H15 expression in wild type, salm KD, and H15 KD flight muscles by immunofluorescence (Fig. S 18 ). As mentioned above, salm KD resulted in a loss of Salm expression (Fig. S 7 , Fig. S 20y ), and H15 KD led to a reduction in H15 expression (Fig. S 20f, z ) in flight muscles as expected. While salm KD in flight muscle led to a decrease in H15 protein and mRNA expression (Fig. S 18v, z, z ’), thereby providing validation to our proteomic findings; H15 KD had no effect on Salm expression in the flight muscles (Fig. S 18n, y ) consistent with H15 regulation of muscle fiber type specification occurring downstream of salm . To provide confirmation of H15 operating downstream of salm in Drosophila muscle, we performed rescue experiments where we overexpressed H15 in the salm KD background (Fig. 5 and Fig. S 19 ). Overexpression of H15 together with salm KD ( H15 OE; salm KD ) did not rescue the flightless phenotype caused by the loss of salm (Fig. S 5a ). However, H15 OE; salm KD did successfully rescue the fibrillar contractile type of the flight muscles from the tubular contractile type observed in salm KD flight muscles (Fig. 5a, e, i ) in 38% of the muscle fibers observed ( n = 26) (Fig. 5m ). Salm expression remained undetectable by immunofluorescence in the fibrillar H15 OE; salm KD flight muscles (Fig. 5a–l, n ) indicating that the contractile type rescue was indeed mediated by H15 . Moreover, mitochondrial networks (assessed with MitoTracker Red) in the rescued H15 OE; salm KD flight muscles also returned to their wild-type, parallel phenotype (Fig. 5o–r ), indicating that H15 can regulate mitochondrial network configuration in flight muscles in the absence of salm . This H15 OE rescue of the salm KD phenotype is not due to GAL4 dilution as the salm KD phenotype is retained in the presence of two UAS ( UAS-salm RNAi::UAS-mito-GFP , Fig. 2f–h ). Overall, these data demonstrate that H15 regulates muscle fiber type specification downstream of salm . Fig. 5: H15 is downstream of salm and H15 OE rescues fiber-type switching in salm KD fibers. a – d Wildtype fibrillar IFM stained for F-actin (phTRITC), nuclei (DAPI), and Salm antibody showing Salm expression in the nuclei. e – h salm KD IFM showing decreased expression of salm and fiber type switch in IFM from fibrillar to tubular. i – l H15 OE; salm KD shows fibrillar fiber type in IFMs and decreased Salm antibody immunofluorescence (Scale Bars: 5 μm for all). m Quantification of fluorescence intensity of Salm antibody staining (Wildtype, n = 12, 3 animals; salm KD, n = 11, 3 animals; H15 OE; salm KD, n = 11, 4 animals). Each point represents the value for each dataset (Wildtype, n = 16; salm KD ( UAS-salm RNAi;UAS-mito-gfp;mef2) (, n = 20 animals; H15 OE; salm KD, n = 26 animals). n Quantification of fiber type in IFMs (Wildtype, n = 16; salm KD ( UAS-salm RNAi;UAS-mito-gfp;mef2) ( n = 20; H15 OE; salm KD, n = 26). o Wildtype IFM showing a parallel mitochondrial network (MitoTracker). p Knockdown of salm (UAS-salm RNAi;UAS-mito-gfp;mef2) in flight muscles coverts parallel mitochondrial arrangement to a grid-like network. q H15 OE; salm KD shows parallel mitochondrial networks in IFMs similar to wildtype (Scale Bars: 5 μm for all). r Quantification of mitochondrial network orientation. Dotted line represents parallel equal to perpendicular (WT IFM, n = 3 animals; salm KD IFM, n = 3 animals; H15 KD; salm OE IFM, n = 3 animals). Each point represents value for each animal dataset. Bars represent mean ± SD. Significance determined as p < 0.05 from one way ANOVA with Tukey’s (*, p ≤ 0.05; **, p ≤ 0.01; ***, p ≤ 0.001; ****, p ≤ 0.0001; ns, non-significant). Full size image cut regulates mitochondrial network organization To identify additional regulators of mitochondrial network organization and/or contractile type in Drosophila muscle, we focused on the transcription factors in addition to H15, which were associated with at least one muscle specification phenotype in our proteomic screen. Of the 142 candidate proteins, six additional transcription factors (Prospero, Limpet, Reversed polarity, cut, CG17822, and CG12605) were identified using the Drosophila Transcription Factor Database [84] including three salm- proteins (Prospero, Reversed polarity, and Limpet) and one each for Fibrillar + (CG12605), Grid + (Limpet), Grid- (CG17822), and Parallel- (cut). We generated flies with muscle-specific ( Mef2-Gal4 ) KD or OE for three of these proteins (Prospero, Limpet, and cut) to determine their potential role in muscle fiber type specification. Limpet is a LIM domain protein that expresses different isoforms in fibrillar and tubular muscles with its splicing pattern regulated by salm [85] . Our proteomic analysis detected four different isoforms of Limpet (A, J, K, and N) (Supplemental Data 1 ) with isoforms A and P both being identified as Grid+ and Salm- proteins (Supplemental Data 2 ) consistent with expression of these isoforms being highest in the leg (Supplemental Data 1 ). Thus, we hypothesized that Limpet KD would alter the mitochondrial network and/or contractile type in the legs whereas Limpet OE would have the greatest effect on the flight muscles. However, Limpet KD flies appeared to fly normally and showed no changes in mitochondrial network configuration or contractile type in the flight, jump, or leg muscles (Fig. S 20 ). Additionally, Limpet OE flies also showed the wild-type mitochondrial network and contractile phenotypes across each muscle group (Fig. S 21 ), though these flies displayed weak flight behavior. These data suggest that while Limpet expression is associated with muscle type, Limpet itself does not regulate the configuration of contractile or mitochondrial networks in Drosophila muscle. Prospero is a homeobox transcription factor critical for neurogenesis and motor neuron innervation in Drosophila muscle [86] , [87] . Additionally, loss of the mammalian ortholog of Prospero, Prox1, in striated muscle leads to an upregulation of fast-twitch contractile proteins in both the heart and skeletal muscle of mice [88] , [89] , and Prox1 directly interacts with ERRα and PGC-1α to negatively modulate their activity in mouse liver cells [90] . Thus, we hypothesized that Prospero would regulate both contractile and mitochondrial network type in Drosophila muscles. Knockdown of Prospero throughout muscle development ( Mef2-Gal4 ) was lethal consistent with the known essential role of its ortholog, Prox1, in myoblast differentiation [89] . Prospero KD from the third instar larval stage ( Tub-Gal80; ts Mef2-Gal4 ) allowed flies to reach adulthood though they remained flightless. Despite the loss of overall muscle function with Prospero KD, the mitochondrial and contractile networks in the flight, jump, and leg muscles retained their wild-type phenotypes, respectively (Fig. S 22 ). Due to the identification of Prospero as a Salm- protein in our proteomic screen, we hypothesized that Prospero OE would convert the contractile and/or mitochondrial networks in the flight muscles. However, flies with muscle-specific overexpression of Prospero maintained parallel mitochondrial networks and fibrillar myofibrils similar to wild-type flight muscles (Fig. S 23 ) albeit with weak flight ability. Thus, despite its indispensable role for normal muscle development and function, these results indicate Prospero does not regulate contractile or mitochondrial network configuration in Drosophila muscles. cut encodes a homeobox transcription factor involved in cell-type specification and patterning across Drosophila organ systems [91] , [92] , [93] , [94] . In muscle, cut expression level is known to differentiate between which third instar wing disc myoblasts will eventually form the fibrillar indirect flight muscles (low cut) or the tubular direct flight muscles (DFM, high cut) [95] , [96] . However, the role of cut in the development of contractile networks in muscles derived from outside the third instar proximal wing imaginal disc (e.g., jump or leg muscles) or in the specification of mitochondrial network type remains unclear. Due to the known role of cut in DFM specification, we first assessed mitochondria in the wild-type DFMs by FIB-SEM which revealed mitochondrial networks arranged in sheets parallel to the tubular contractile networks (Fig. S 24 ) suggesting that cut regulates contractile type, but not the orientation of mitochondrial networks in DFMs. Since our proteomic analyses identified cut as a Parallel-protein (Supplemental Data 2 ), we hypothesized that cut KD would alter the grid-like mitochondrial networks in the leg muscles and that cut OE would affect the parallel mitochondrial networks in the flight and jump muscles. Muscle-specific (Mef2-Gal4) cut KD permitted development to adulthood, but with a complete loss of flight activity and weak climbing ability compared to wild-type flies (Fig. S 5a, b ). We were unable to detect cut by immunofluorescence in wild-type adult muscles, so muscle-specific cut KD was confirmed by the loss of cut immunofluorescence in Mef2-positive third instar proximal wing imaginal disc cells (Fig. S 26 ). Flight and jump muscle contractile and mitochondrial networks were unaffected by cut KD (Fig. S 27 ), as were the contractile networks in the leg muscles (Fig. S 28a, d, g, j ). However, while the mitochondrial networks in Fibers I and III of the cut KD legs retained the wild-type parallel and grid-like configurations, respectively (Fig. 6a, b and Fig. S 28a–l ), the mitochondrial networks in Fiber II of the cut KD leg were converted from grid-like to parallel (Fig. 6d, g, i ) (Supplementary Movie 8 ) in 78.6% of the muscles assessed ( n = 14) (Fig. S 28m ) without a change in mitochondrial content (Fig. 6j ). These results indicate that cut regulates mitochondrial network configuration, independent of contractile fiber-type, in a regionally specific manner within the leg muscles. Fig. 6: cut regulates conversion of mitochondrial networks configuration, but not contractile type, in Fiber II of Drosophila leg muscles. a Adult wildtype leg coxa muscles showing distinct parallel and grid-like mitochondrial networks (mito-gfp) in Fiber I, II, and III (demarcated by dotted lines). b cut KD converts grid-like mitochondrial networks to parallel in Fiber II (Scale Bars: 20 μm). c , d Wildtype leg Fiber I showing parallel mitochondrial networks (mito-GFP) and tubular muscle fiber (phTRITC). e , f Wildtype leg Fiber II and g , h Fiber III showing grid-like mitochondrial networks (mito-GFP) and tubular muscle fiber (phTRITC). i , j cut KD Fiber I showing parallel mitochondrial networks (mito-GFP) and tubular muscle fiber (phTRITC). k , l cut KD Fiber II showing parallel mitochondrial networks (mito-GFP), unlike wildtype Fiber II, while fibers remain tubular (phTRITC). m , n cut KD Fiber III showing grid-like mitochondrial networks (mito-GFP) and tubular muscle fibers (phTRITC). (Scale Bars: 5 μm for all). o Quantification of mitochondrial network orientation. Dotted line represents parallel equal to perpendicular. mito-gfp;mito-mcherry;mef2-Gal4 used as Wildtype, WT (WT-Fiber I, n = 4 animals; cut KD-Fiber I, n = 4 animals; WT-Fiber II, n = 3 animals; cut KD-Fiber II, n = 6 animals; WT-Fiber III, n = 4 animals; cut KD-Fiber III, n = 4 animals). p Mitochondrial volume as a percent of total muscle volume. UAS-mito-gfp;UAS-mitoOMM-mcherry;mef2-Gal4 used as wildtype (WT-Leg Fiber I, n = 4 animals; cut KD-Leg Fiber I, n = 7 animals; WT-Leg Fiber II, n = 4 animals; cut KD-Leg Fiber II, n = 10 animals; WT-Leg Fiber III, n = 5 animals; cut KD-Leg Fiber III, n = 5 animals). Each point represents value for each animal dataset. Bars represent mean ± SD. Significance determined as p < 0.05 from one way ANOVA with Tukey’s (*, p ≤ 0.05; **, p ≤ 0.01; ***, p ≤ 0.001; ****, p ≤ 0.0001; ns, non-significant). Full size image To identify whether cut operates in the same mitochondrial network configuration specification pathway as salm and H15 , we further investigated the relationship between cut and salm . Expression of cut protein was increased above wild type levels in both the salm KD flight muscles and the salm OE leg muscles (Supplemental Data 1 ) suggesting that salm does not regulate the expression of cut . Indeed, cut and transcription factor vestigial are known to act in a mutually repressive fashion [95] , and salm expression in flight muscles has been shown to require upstream expression of vestigial [67] , suggesting that cut may act as an upstream repressor of salm . To test this hypothesis, we investigated whether combining cut KD and salm KD ( cut KD; salm KD) would rescue the contractile and mitochondrial network phenotypes observed in salm KD flight muscles. While cut KD; salm KD flies were unable to fly (Fig. S 5a ), the flight muscle contractile networks were fibrillar and the mitochondrial networks were parallel similar to the wild type flight muscles (Fig. 7d–f ). Further, significant Salm immunofluorescence was detected in the cut KD; salm KD flight muscles (Fig. 7q ) indicating that Salm may no longer be knocked down sufficiently to induce a fiber type transformation. To investigate this possibility, we performed qPCR analysis of salm transcript levels in the flight muscles of wild type, salm KD, cut KD, and cut KD; salm KD flies. Though salm KD resulted in an ~60% decrease in salm transcript expression relative to wild-type flies, there was no difference in salm expression between wild type and cut KD; salm KD flight muscles (Fig. 7s ) indicating that salm was no longer knocked down upon the addition of cut KD. The rescue of salm expression in the cut KD; salm KD flight muscles was not due to GAL4 dilution in the presence of a second UAS ( UAS-salm RNAi::UAS-cut RNAi ) since salm KD mediated flight muscle conversion still occurs with two UAS ( UAS-salm RNAi::UAS-mito-GFP , Fig. 2f–h ). Further, salm transcript levels were increased ~60% above wild type levels in the cut KD flight muscles (Fig. 7s ) indicating that the increase in salm expression in the cut KD; salm KD flight muscles relative to the salm KD flight muscles was indeed mediated by cut . Fig. 7: cut is a repressor of salm and cut KD rescues fiber-type switching and conversion of mitochondrial network organization in salm KD fibers. a , b , c Fibrillar flight muscles (IFMs) stained for F-actin (phTRITC) and mitochondria (MitoTracker) showing parallel aligned mitochondria between myofibrils. d , e , f salm KD ( UAS-salm RNAi;UAS-mito-gfp;mef2) shows fibrillar muscles switched to tubular muscle type and mitochondria (mito-gfp) converted to grid-like networks. g , h , i salm KD; cut KD shows fibrillar fiber type and parallel mitochondrial networks (MitoTracker) in IFMs similar to wildtype. j , k , l cut -OE shows tubular fiber type and grid-like mitochondrial networks (MitoTracker) in IFMs similar to salm KD ( UAS-salm RNAi;UAS-mito-gfp;mef2) (Scale Bars: 5 μm for all). m Quantification of mitochondrial network orientation. Dotted line represents parallel equal to perpendicular (WT IFM, n = 3 animals; salm KD( UAS-salm RNAi;UAS-mito-gfp;mef2) IFM, n = 3 animals; salm KD; cut KD IFM, n = 3 animals ; cut-OE, n = 4 animals). n Wildtype fibrillar IFM stained for nuclei (DAPI), and salm antibody showing salm expression in the nuclei. o salm KD IFM showing decreased salm expression. p cut KD IFM and q salm KD; cut KD showing restored salm expression in the nuclei. r cut -OE showing absence of salm expression in the nuclei (Scale Bars: 5 μm for all). s Quantification of salm transcript levels (WT IFM, n = 5; salm KD ( UAS-salm RNAi;UAS-mito-gfp;mef2) IFM, n = 5; cut KD, n = 3; salm KD; cut KD IFM, n = 3 ). t Quantification(qPCR) of cut , salm, and H15 transcript levels. Each point represents value for each dataset. Bars represent mean ± SD. Significance determined as p < 0.05 from one way ANOVA with Tukey’s (*, p ≤ 0.05; **, p ≤ 0.01; ***, p ≤ 0.001; ****, p ≤ 0.0001; ns, non-significant). Full size image To further test the hypothesis that cut operates upstream of salm , we assessed the impact of cut OE on contractile and mitochondrial network configuration and salm expression. Muscle-specific (Mef2-Gal4 driven) overexpression of cut resulted in 100% pupal lethality and precluded phenotypic analyses of adult flight and jump muscles. However, flight muscle-specific ( Act88f -Gal4 and 1151 -Gal4 driven) overexpression of cut , confirmed by qPCR (Fig. 7t ), allowed adult flies to eclose and resulted in tubular flight muscles with centralized nuclei and grid-like mitochondrial networks similar to those observed in salm KD flight muscles (Fig. 7j–l,m , Fig. S 25 ). Moreover, both Act88f -Gal4 and 1151 -Gal4 driven cut OE resulted in a loss of Salm protein and transcript expression compared to wild-type flight muscles (Fig. 7n–r, t , Fig. S 25 ) similar to the reductions observed in salm KD flight muscles (Fig. S 7o , Fig. 7s ). Additionally, Act88f -Gal4 driven cut OE led to a reduction in H15 transcript expression whereas the 1151 -Gal4 driven loss of H15 expression due to cut OE did not reach significance (Fig. 7t ). Overall, these data demonstrate that cut operates as an upstream repressor of salm capable of regulating contractile and mitochondrial network configuration in a muscle-specific manner. Muscle contraction is an energetically demanding process occurring in a tightly packed cellular environment, thereby requiring close coordination between the architectures of the contractile and metabolic machineries to optimally support the function the muscle cell. While regulation of metabolic and contractile properties occurs together early in the muscle-type specification process [37] , [97] , [98] , at which point(s) the regulation of mitochondrial network structure diverges into a pathway independent from contractile network structure is not well understood. Here, we utilized the naturally occurring functional differences among Drosophila muscles [61] , [63] combined with the known Drosophila muscle type specification factor salm to identify 142 proteins consistently associated with either fibrillar or tubular contractile types, parallel or grid-like mitochondrial networks, or salm expression level. By performing phenotypic assessments of the contractile and mitochondrial networks in the flight, jump, and leg muscles of flies with knockdown or overexpression of five additional transcription factors identified by our screen, we demonstrate that mitochondrial network configuration and contractile type can be regulated independently through evolutionarily conserved transcription factors cut , salm , and H15 . Moreover, we show that the regulatory role of each of these transcription factors for mitochondrial network specification can be variable among the flight, jump, and leg muscles and even within different regions of the leg muscles. The parallel mitochondrial networks running between the fibrillar myofibrils of the flight muscles can be converted to grid-like mitochondrial networks reminiscent of the tubular leg muscles in the absence of salm as shown here (Fig. 2g ) and elsewhere [50] while the current paper was under revision. Further, we find here that salm regulation of mitochondrial network configuration in flight muscles is mediated by downstream regulator H15 as H15 overexpression in the absence of salm is sufficient to restore the flight muscles back to their wild-type parallel mitochondrial network phenotype (Fig. 5n–p ). However, loss of H15 alone resulted in the conversion of the flight muscles to a jump muscle phenotype with parallel mitochondrial networks located within a tubular contractile network (Fig. 4d, e ). Thus, conversion of the contractile network of the flight muscles from fibrillar to tubular can occur with ( salm KD) or without ( H15 KD) conversion of the mitochondrial network highlighting the capacity for independent regulation of the two major structural components within the flight muscle cell. We found that the mitochondrial networks in the tubular muscles can take either a parallel (jump/leg Fiber I) or grid-like (leg Fiber II/III) configuration (Fig. 1 ) again demonstrating the independent nature of the mitochondrial network and contractile type specification processes. Whereas the mitochondrial properties of the flight muscles have been widely studied [46] , [47] , [60] , [99] , there has been relatively little investigation into how metabolism may vary across tubular muscle types. Similar to the differences in mitochondrial content we have shown here among tubular muscles (Fig. 1t ), two different levels of mitochondrial enzyme activity within the leg muscles, each higher than the activity of the jump muscle, has been reported previously [65] . However, the flight muscle, jump muscle, and Fiber I of the leg all have parallel mitochondrial networks despite largely different mitochondrial contents (Fig. 1u ) and enzyme activity levels [65] suggesting that mitochondrial network configuration may be specified differently than mitochondrial content. Indeed, we find that H15 KD converts the parallel mitochondrial networks of the jump and leg Fiber I muscles to more grid-like networks (Fig. 4 ) and cut KD converts the grid-like mitochondrial networks in Fiber II of the leg to parallel (Fig. 6 ) each without altering mitochondrial content (Fig. 6j and Fig. S 14b ) or the tubular nature of the myofibrils. Thus, regulation of mitochondrial network configuration also appears to occur independently from mitochondrial content and enzyme activity in addition to contractile type. A separation of the mitochondrial content and network configuration specification processes may also explain why loss of spargel , the Drosophila PGC-1α ortholog, does not alter the location of mitochondria between the myofibrils in flight muscles despite having a significant effect on individual mitochondrial structure and metabolism [15] . Mitochondrial dynamics proteins governing the capacity for mitochondrial fission, fusion, and motility have been shown to regulate the structure of individual mitochondria, mitochondrial network formation, and/or maintenance of mitochondrial quality control across a variety of cell types [20] , [22] , [74] , [75] , [76] , [77] . However, consistent with images from previous studies in the flight muscle, we found that loss of Marf (mfn1/2 ortholog) [46] , [47] , [48] , [49] , [50] , Drp1 [52] , Fis1 [53] , and Miro [54] did not change the parallel configuration of mitochondrial networks in the fibrillar muscles despite each gene modulating individual mitochondrial size (Fig. S 4 ). Moreover, overexpression of both Drp1 and Miro has also been shown to alter mitochondrial size, but not network configuration in Drosophila flight muscles [50] , [55] . Thus, these data indicate that regulation of individual mitochondrial size by mitochondrial dynamics proteins can occur independently from specification of mitochondrial network configuration. It should be noted that Mef2-Gal4 driven overexpression of Marf and expression of a dominant negative (DN) form of Drp1 were both found recently to cause conversion of the flight muscles to a tubular contractile apparatus [50] . However, the effects of Marf OE and DN- Drp1 on flight muscle mitochondrial networks appeared variable across the images provided, and neither individual mitochondrial size nor network orientation were quantified precluding direct comparisons. What is clear from the available Marf OE and DN- Drp1 data [50] is that the flight muscle mitochondrial networks did not take a grid-like configuration as seen in the wild-type leg muscles or salm KD flight muscles and instead appeared to vary between the wild-type phenotypes of the tubular DFM and jump muscles, which both have parallel mitochondrial network configurations despite the large increase in mitochondrial size and content in the DFMs. Thus, these data are consistent with the capacity of Drosophila muscles to regulate both contractile type and mitochondrial size separately from mitochondria network configuration as shown here. We propose that the specification of mitochondrial network configuration is an independent process within the overall cellular design of the muscle cell. Through assessment of the contractile and mitochondrial networks in the flight, jump, and leg muscles of flies expressing wild-type, increased, and/or decreased levels of nine genes associated with mitochondrial dynamics or muscle contractile type, we find that mitochondrial network configuration, mitochondrial content, individual mitochondrial size, and contractile type can each be modulated without affecting the other parameters thereby demonstrating the independent nature of each of these aspects of muscle cell design. As shown here, the pathway regulating muscle mitochondrial network configuration involves cut upstream from salm and H15 downstream from salm (Fig. S 29 ). However, additional factors are likely involved. Indeed, transcription factors extradenticle ( exd ) , homothorax ( hth ), and vestigial ( vg ) are each known to specify muscle cell fate upstream from salm [50] , [67] , [78] , [95] . Moreover, vertebrate orthologs of exd (Pbx1-4), hth (Meis1-4), vg (Vgll1-3), and H15 (Tbx15) have all been shown to play a role in muscle fiber type specification [81] , [100] , [101] , [102] indicating that the specific regulation of mitochondrial network configuration as shown here is likely an evolutionarily conserved process, although the specific roles of salm (sall1-4) and cut (cux1–2) orthologs have yet to be determined in mammalian striated muscles. Drosophila strains and genetics Genetic crosses were performed on yeast corn medium at 25 °C unless mentioned. W 1118 were used as controls and respective genetic backgrounds. 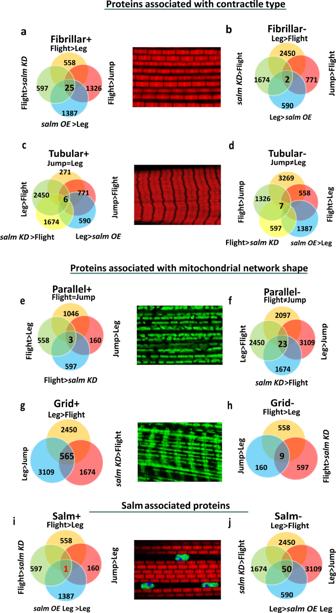Fig. 3: Identification of potential regulatory factors for contractile and mitochondrial network type in Drosophila muscle. aVenn diagram displaying the individual muscle group comparisons and their overlap for proteins positively associated with fibrillar muscles.bVenn diagram displaying the individual muscle group comparisons and their overlap for proteins negatively associated with fibrillar muscles.c,dVenn diagram for tubular positively and negatively associated proteins, respectively.e,fVenn diagram for positively and negatively associated proteins, respectively, with parallel mitochondrial networks.g,hVenn diagram for positively and negatively associated proteins, respectively, with grid-like mitochondrial networks.i,jVenn diagram forsalmpositively and negatively associated proteins, respectively. Both males and females were used and grouped together due an observed lack of sex differences in mitochondrial network configuration in wild type muscles. Mef2- Gal4 (III) was used to drive muscle specific gene knockdown and over expression of respective genes. Tub-Gal80; ts Mef2 Gal4 used for ectopic expression of salm in muscles. UAS-mito-GFP (II chromosome BS# 8442) was used for mitochondrial network visualization. UAS- mito-mcherry (III) was used for visualization of the outer mitochondrial membrane. UAS- H15 RNAi trip lines were used for muscle specific knock down of H15 gene. UAS-mito-mcherry (BS# 66533), Mef2 -Gal4 (BS# 27390), Act88F-Gal4 (III, BS# 38461), 1151-Gal4 [103] , [104] (I, gift from Dr. Upendra Nongthomba) UAS-H15 RNAi (V28415), UAS-Drp1RNAi (BS# 51483) , Marf RNAi (BS# 55189), UAS- salm (Dr. Frank Schnorrer), UAS-salm RNAi (V101052), UAS-Miro RNAi (V106683), UAS-Fis1 RNAi (BS# 63027), UAS-cut RNAi (BS# 33967, #29625), UAS-H15/nmr1 (Dr. Rolf Bodmer), UAS- cut [105] (gift from Dr. Yuh Nung Jan, UCSF, USA), cut-OE (TOE.GS00041) (BS# 67524), UAS-Cas9.P2; Mef2-GAL4 /TM6B, (BS# 67075), UAS-dCas9/cyO; Mef2-GAL4 (BS# 67041), H15-OE (BS# 78722) [106] , UAS-RFP.KDEL (BS# 30910, # 30909) (Dr. Richa Rikhy), Zasp52MI02908-mCherry [107] (Dr. Frieder Schöck). UAS-pros ORF (F004799, FlyORF), UAS- pros RNAi (BS# 26745), UAS-Lmpt.ORF.3xHA . (F001889), UAS-Lmpt RNAi (v105170, 100716). All other stocks were requested or obtained from the VDRC (Vienna) Drosophila stock center, Bloomington (BS#) Drosophila stock center or FLYORF (Zurich) Drosophila stock center. All chromosomes and gene symbols are as mentioned in Flybase ( http://flybase.org ). Mitochondrial networks staining of flight (IFM), jump(TDT), and leg muscles 2–3-day-old adult Drosophila thoraces were dissected in 4% paraformaldehyde (PF, Sigma) with fine scissors, isolating each muscle type: IFMs, jump muscles (TDT) and leg muscles. IFMs, TDT, leg muscles were fixed in 4% PF for 2 h, 1.5 h, and 1.5 h, respectively using a rotor then washed in PBSTx (PBS + 0.3% TritonX100) thrice each for 15 min. Mitochondrial staining dyes (Mito Tracker Red (M22425, Thermofisher, USA) and Acridine Orange nonyl bromide (A7847, Sigma, USA) or DMef2-Gal4 driven UAS-mito-GFP or UAS-mito OMM-mcherry were used to image mitochondrial networks. Actin staining was performed by incubating 2.5 µg/ml of Phalloidin in PBS (Sigma, 1 mg/ml stock of Phalloidin TRITC) at 25 °C for 40 min for IFMs, 20 min for jump muscles and 1 h for leg muscles at RT, respectively. Tissues were mounted on a glass slide with Prolong Glass Antifade Mountant with NucBlue stain (P36985, Thermofisher, USA) and images were captured with Zeiss 780 confocal microscope. Immunohistochemistry Fly thoraces were dissected for IFMs, jump muscles (TDT) and leg muscles in 4% PF and were processed as mentioned Rai et al. [47] . Briefly, each muscle group was fixed in 4% PF; thoraces with IFMs for 2 h, jump muscles for 1.5 h, and leg muscles for 1–1.5 h at room temperature (25 °C, RT) on a rotor. Samples were washed three times with PBSTx (PBS + 0.03% Triton X-100) for 15 min and blocked for 2 h at RT or overnight at 4 °C using 2% BSA (Bovine Serum Albumin, Sigma). Samples were incubated with respective primary antibody (Ab) at 4 °C overnight and later washed three times for 10 min with PBSTx and incubated for 2.5 h in respective secondary Ab at 25 °C or overnight at 4 °C. Samples were incubated for 40 min with Phalloidin TRITC (2.5 µg/ml) (P1951, Sigma, USA) to counter stain samples and mounted using Prolong Glass Antifade Mountant with NucBlue stain and incubated for 20 min. Images were acquired with Leica SP8 STED 3X/Confocal Microscope and ZEISS 780 confocal microscope and processed using ImageJ and ZEN software (version 3.2.0.115) respectively. 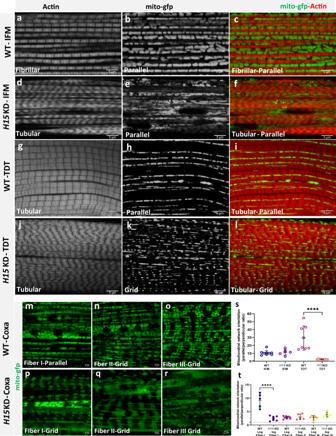Fig. 4:H15independently regulates the conversion of muscle contractile type and mitochondrial network configuration in Drosophila muscles. a,b,cFibrillar flight muscles (IFMs) stained for F-actin (phTRITC) and mitochondria (mito-GFP) showing parallel aligned mitochondria between myofibrils.dH15KD shows fibrillar muscles switched to tubular muscle type.e,fH15KD muscles show parallel mitochondria along muscle fibers.g,h,iTubular jump muscles show parallel mitochondria (thin and elongated).jH15KD in jump muscles shows tubular fibers (phTRITC).k,lUponH15KD, tubular jump muscles show a change in mitochondrial networks to more grid-like (Scale Bars: 5 μm for all).mWildtype coxa leg muscle Fiber I showing parallel mitochondrial networks.nWildtype leg muscle Fiber II andoFiber III showing grid-like mitochondrial networks.pH15KD leg muscle Fiber I showing conversion to a grid-like mitochondrial network.q,rH15KD leg muscle fibers II and III show grid-like structures similar to their wild type counterparts (Scale Bars: 5 μm for all).sQuantification of mitochondrial network orientation. Dotted line represents parallel equal to perpendicular.mito-gfp;mito-mcherry;mef2-Gal4used as wildtype, WT; indirect flight muscles, IFM; Jump muscles, TDT. (WT-IFM,n=9animals;H15KD-IFM,n=6animals; WT-TDT,n=8animals;H15KD-TDT,n=8animals).tQuantification of mitochondrial network orientation in leg (walking) Fibers. (WT-leg Fibers I,n=5animals;H15KD-IFM,n=7animals; WT-leg Fiber II,n=9animals;H15KD-Leg Fiber II,n=5animals; WT-Leg Fiber III,n=6animals,H15KD-Leg Fiber III,n=5animals). Each point represents value for each dataset. Bars represent mean ± SD. Significance determined asp< 0.05 from one way ANOVA with Tukey’s (*,p≤ 0.05; **,p≤ 0.01; ***,p≤ 0.001; ****,p≤ 0.0001; ns, non-significant). Antibodies used for the staining: Rabbit anti-salm-1 (1:500, gift from Dr. Tiffany Cook [108] ,), Rabbit anti-nmr1 (H15) (1:200, gift from Dr. James B. Skeath [109] ,), Mouse anti-cut (1:20, 2B10, DHSB), Alexa Fluor 594-labeled Goat anti-Mouse IgG (1:500, Cat# A-11032) and Alexa-Fluor-488-labeled anti-rabbit IgG (1:500, Cat# A32731, Thermofisher, USA). The mean fluorescence intensity of antibody immunostaining was measured as reported previously [110] using ImageJ. Three-dimensional rendering of mitochondria networks was performed using IMARIS 9.7.0 ( http://www.bitplane.com/imaris/imaris ). Real-time quantitative PCR Total RNA was extracted from thorax muscles of 1–2 day-old adult flies using the TRIzol™ Plus RNA Purification Kit (A33254) according to the manufacturer’s instructions. DNA digestion was carried out using TURBO DNA-free™ Kit (AM1907) and first-strand synthesis was performed using 500 ng of total RNA using SuperScript™ VILO™ cDNA Synthesis Kit (Thermo Fisher Scientific, 11754050). Standard curves were generated using concentrated cDNA from all samples. Amplification was detected on the QuantStudio3 Real-Time PCR System (Thermo Fisher Scientific). RLP32 reference gene was used for normalization and reactions were performed in triplicates. The TaqMan Probes salm (Assay ID: Dm01804248_g1), cut (Assay ID: Dm01837171_m1) H15 (Assay ID: Dm01804677_m1), fln (Assay ID:Dm01823176_g1), Act88F (Assay ID:Dm02362815_s1), TpnC4 (Assay ID:Dm01815264_m1) and RLP32 (Assay ID: Dm02151827_g1) were used. Behavioral assays Flight test The flight was assayed at room temperature (22 °C) using a flight box, as detailed earlier [46] , [47] . Two to three-day-old flies were independently scored for flight ability as up flighted (U), horizontally flighted (H), down flighted (D), or flightless (F). Each fly was tested thrice. Jump test Jump tests were performed for the 2–3 days old adult flies as described previously [111] . Adult fly wings were removed and flies were allowed to recover for 24 h at room temperature (RT). Then, the flies were placed on a platform raised above a sheet of white paper and encouraged to jump from the platform using a paintbrush. The point of landing on the paper was marked and the distances were measured from the edge of the platform to the marked point in mm. Each fly was tested thrice and the average jump distance was calculated. Climbing assay Two–three-day-old flies were divided into three groups of ten flies in each vail and allowed to recover. Climbing assay was performed as previously described [112] . Groups of ten flies were placed in an empty climbing vial and then tapped down to the bottom. They were allowed 18 s to climb up to a line marked 5 cm from the bottom of the vial. The number of flies above the 5 cm mark at 18 s was recorded as the percentage of flies able to climb. Image analysis and quantifications Individual mitochondrial area and aspect ratio Individual mitochondria were traced using the freehand tool of ImageJ software ( https://imagej.net ) on 2D light microscopic images. Individual mitochondrial area and aspect ratio (ratio of major axis/minor axis) were calculated using ImageJ software [46] . Mitochondrial and ER content Light microscopic images were opened using ImageJ and binarized and the total mitochondrial volume was determined as the percentage of binarized mitochondrial pixels per total muscle fiber pixels. ER content was calculated as the percentage of binarized ER pixels per total muscle fiber pixels Mitochondrial network analysis Mitochondrial network analysis was performed as described using ImageJ software [31] . The mitochondrial network orientation analysis was performed on 2D images, where the mitochondrial image was rotated such that the horizontal axis was parallel to the direction of muscle contraction. The images were then binarized and the OrientationJ Distributions plugin was used to determine the angles of the mitochondrial network. Parallel mitochondria were determined as those with a ±0–10° angle to the axis of muscle contraction and perpendicular mitochondria were determined as those with a ± 80–90° angle to the axis of muscle contraction. Proteomic analysis Drosophila muscle protein extraction Three to four days old Drosophila thoraces were chopped soon after freezing in liquid nitrogen and each muscle type dissected (IFMs(n100), Jump muscles ( n = 200) -TDT and Leg muscles ( n = 250-300), salm KD IFMs ( n = 200) salm OE leg muscles ( n = 25–300) in 70% alcohol. Muscle protein extraction preparation was followed as described in Kim et al., 2019. Muscle tissues were transferred to 90 µl of urea-based lysis buffer (6 M Urea, 2 M Thiourea, 50 mM Triethylammonium bicarbonate [TEAB]) at 1:5 ratio. Tissues were homogenized with ceramic beads using three steps of 45 s at 6500 rpm and 4 °C (Precellys® Cryolys Evolution, Bertin Technologies). Legs were sonicated for 30 s twice for better homogenization and muscle samples were collected. Tissue lysates were further homogenized and centrifuged at 10,000 g for 10 min at 4 °C in microcentrifuge spin columns (QIAshredder, Qiagen) to obtain clear protein lysate. The extracted protein supernatants were transferred to 1.5 ml microtubes for further processing. Protein concentration was estimated by Bradford assay (ThermoFisher Scientific). Briefly, 100 µg of each sample was digested with trypsin, labeled with Tandem Mass Tag (TMT) 11plex labeling reagent kit following manufacturer’s instructions (Thermo Fisher Scientific), quenched with 5% hydroxylamine, and combined to make a total of 1 mg in a single microcentrifuge tube. The combined samples were desalted using a 1 cc Oasis HLB cartridge (Waters) following manufacturer’s instructions and speedvaced to dryness. Offline HPLC peptide fractionation High pH reversed-phase liquid chromatography was performed on an offline Agilent 1200 series HPLC. Approximately, 1 mg of desalted peptides were resuspended in 0.1 ml 10 mM triethyl ammonium bicarbonate with 2% (v/v) acetonitrile. Peptides were loaded onto an Xbridge C 18 HPLC column (Waters; 2.1 mm inner diameter × 100 mm, 5 μm particle size), and profiled with a linear gradient of 5–35% buffer B (90% acetonitrile, 10 mM triethyl ammonium bicarbonate[TEAB]) over 60 min, at a flowrate of 0.25 ml/min. The chromatographic performance was monitored by sampling the eluate with a diode array detector (1200 series HPLC, Agilent) scanning between wavelengths of 200 and 400 nm. Fractions were collected at 1 min intervals followed by fraction concatenation. Fifteen concatenated fractions were dried and resuspended in 0.01% formic acid, 2% acetonitrile. Approximately 500 ng of peptide mixture was loaded per liquid chromatography-mass spectrometry run. Mass spectrometry All fractions were analyzed on an Ultimate 3000-nLC coupled to an Orbitrap Fusion Lumos Tribrid instrument (Thermo Fisher Scientific) equipped with a nanoelectrospray source. Peptides were separated on an EASY-Spray C 18 column (75 μm × 50 cm inner diameter, 2 μm particle size and 100 Å pore size, Thermo Fisher Scientific). Peptide fractions were placed in an autosampler and separation was achieved by 120 min gradient from 4 to 24% buffer B (100% ACN and 0.1% formic acid) at a flow rate of 300 nL/min. An electrospray voltage of 1.9 kV was applied to the eluent via the EASY-Spray column electrode. The Lumos was operated in positive ion data-dependent mode, using Synchronous Precursor Selection (SPS-MS3). Full scan MS1 was performed in the Orbitrap with a precursor selection range of 380–1500 m/z at nominal resolution of 1.2 × 10 5 . The AGC target and maximum accumulation time settings were set to 4 × 10 5 and 50 ms, respectively. MS2 was triggered by selecting the most intense precursor ions above an intensity threshold of 5 × 10 3 for collision induced dissociation (CID)-MS2 fragmentation with an AGC target and maximum accumulation time settings of 2 × 10 4 and 75 ms, respectively. Mass filtering was performed by the quadrupole with 0.7 m/z transmission window, followed by CID fragmentation in the linear ion trap with 35% normalized collision energy in rapid scan mode and parallelizable time option was selected. SPS was applied to co-select ten fragment ions for HCD-MS3 analysis. SPS ions were all selected within the 400–1200 m/z range and were set to preclude selection of the precursor ion and TMTC ion series. The AGC target and maximum accumulation time were set to 1 × 10 5 and 150 ms (respectively) and parallelizable time option was selected. Co-selected precursors for SPS-MS3 underwent HCD fragmentation with 65% normalized collision energy and were analyzed in the Orbitrap with nominal resolution of 5 × 10 4 . The number of SPS- MS3 spectra acquired between full scans was restricted to a duty cycle of 3 s. Data processing Raw data files were processed using Proteome Discoverer (v2.3, Thermo Fisher Scientific), with Mascot (v2.6.2, Matrix Science) search node. The data files were searched against Translated EMBL (TrEMBL) Drosophila melanogaster protein sequence database (uniport.org), with carbamidomethylation of cysteine, TMT 11-plex modification of lysines and peptide N-terminus set as static modifications; oxidation of methionine and deamidation of asparagine and glutamines as dynamic. For SPS-MS3, the precursor and fragment ion tolerances of 10 ppm and 0.5 Da were applied, respectively. 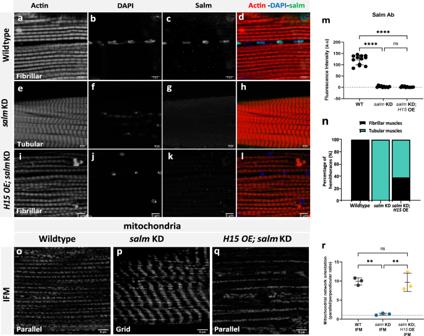Fig. 5:H15is downstream ofsalmandH15OE rescues fiber-type switching insalmKD fibers. a–dWildtype fibrillar IFM stained for F-actin (phTRITC), nuclei (DAPI), and Salm antibody showing Salm expression in the nuclei.e–hsalmKD IFM showing decreased expression of salm and fiber type switch in IFM from fibrillar to tubular.i–lH15 OE;salmKD shows fibrillar fiber type in IFMs and decreased Salm antibody immunofluorescence (Scale Bars: 5 μm for all).mQuantification of fluorescence intensity of Salm antibody staining (Wildtype,n= 12, 3 animals;salmKD,n= 11, 3 animals;H15OE;salmKD,n= 11, 4 animals). Each point represents the value for each dataset (Wildtype,n= 16;salmKD (UAS-salm RNAi;UAS-mito-gfp;mef2)(,n= 20 animals;H15OE;salmKD,n= 26 animals).nQuantification of fiber type in IFMs (Wildtype,n= 16;salmKD (UAS-salm RNAi;UAS-mito-gfp;mef2)(n= 20;H15OE;salmKD,n= 26).oWildtype IFM showing a parallel mitochondrial network (MitoTracker).pKnockdown ofsalm (UAS-salm RNAi;UAS-mito-gfp;mef2)in flight muscles coverts parallel mitochondrial arrangement to a grid-like network.qH15OE;salmKD shows parallel mitochondrial networks in IFMs similar to wildtype (Scale Bars: 5 μm for all).rQuantification of mitochondrial network orientation. Dotted line represents parallel equal to perpendicular (WT IFM,n= 3 animals;salmKD IFM,n= 3 animals;H15KD;salmOE IFM,n= 3 animals). Each point represents value for each animal dataset. Bars represent mean ± SD. Significance determined asp< 0.05 from one way ANOVA with Tukey’s (*,p≤ 0.05; **,p≤ 0.01; ***,p≤ 0.001; ****,p≤ 0.0001; ns, non-significant). Up to two-missed tryptic cleavages were permitted. Percolator algorithm was used to calculate the false discovery rate (FDR) of peptide spectrum matches, set to q value 0.05.TMT 11-plex quantification was also performed by Proteome Discoverer by calculating the sum of centroided ions within 20 ppm window around the expected m/z for each of the 11 TMT reporter ions. Spectra with at least 60% of SPS masses matching to the identified peptide are considered as quantifiable PSMs. Quantification was performed at the MS3 level where the median of all quantifiable PSMs for each protein group was used for protein ratios. Only proteins detected in all samples were included for analysis. A relative protein abundance threshold of greater than or equal to 2.0 or less than or equal to 0.5 was used to determine proteins which were differentially expressed between muscle types and proteins with abundances within 25% were considered of similar abundance. 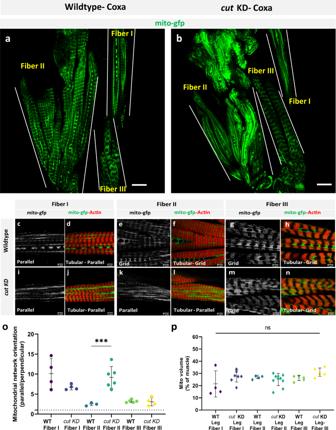Fig. 6:cutregulates conversion of mitochondrial networks configuration, but not contractile type, in Fiber II of Drosophila leg muscles. aAdult wildtype leg coxa muscles showing distinct parallel and grid-like mitochondrial networks (mito-gfp) in Fiber I, II, and III (demarcated by dotted lines).bcutKD converts grid-like mitochondrial networks to parallel in Fiber II (Scale Bars: 20 μm).c,dWildtype leg Fiber I showing parallel mitochondrial networks (mito-GFP) and tubular muscle fiber (phTRITC).e,fWildtype leg Fiber II andg,hFiber III showing grid-like mitochondrial networks (mito-GFP) and tubular muscle fiber (phTRITC).i,jcutKD Fiber I showing parallel mitochondrial networks (mito-GFP) and tubular muscle fiber (phTRITC).k,lcutKD Fiber II showing parallel mitochondrial networks (mito-GFP), unlike wildtype Fiber II, while fibers remain tubular (phTRITC).m,ncutKD Fiber III showing grid-like mitochondrial networks (mito-GFP) and tubular muscle fibers (phTRITC). (Scale Bars: 5 μm for all).oQuantification of mitochondrial network orientation. Dotted line represents parallel equal to perpendicular.mito-gfp;mito-mcherry;mef2-Gal4used as Wildtype, WT (WT-Fiber I,n= 4 animals;cutKD-Fiber I,n=4animals; WT-Fiber II,n=3animals;cutKD-Fiber II,n= 6 animals; WT-Fiber III,n= 4 animals;cutKD-Fiber III,n= 4 animals).pMitochondrial volume as a percent of total muscle volume.UAS-mito-gfp;UAS-mitoOMM-mcherry;mef2-Gal4used as wildtype (WT-Leg Fiber I,n= 4 animals;cutKD-Leg Fiber I,n= 7 animals; WT-Leg Fiber II,n= 4 animals;cutKD-Leg Fiber II,n= 10 animals; WT-Leg Fiber III,n=5animals;cutKD-Leg Fiber III,n=5animals). Each point represents value for each animal dataset. Bars represent mean ± SD. Significance determined asp< 0.05 from one way ANOVA with Tukey’s (*,p≤ 0.05; **,p≤ 0.01; ***,p≤ 0.001; ****,p≤ 0.0001; ns, non-significant). 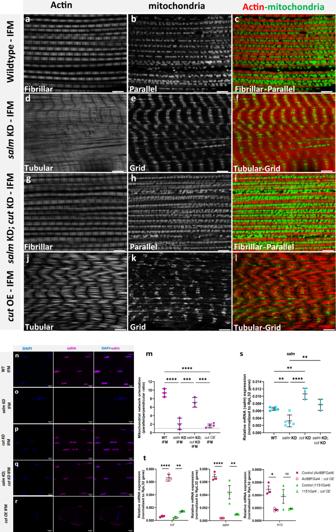Fig. 7:cutis a repressor ofsalmandcutKD rescues fiber-type switching and conversion of mitochondrial network organization insalmKD fibers. a,b,cFibrillar flight muscles (IFMs) stained for F-actin (phTRITC) and mitochondria (MitoTracker) showing parallel aligned mitochondria between myofibrils.d,e,fsalmKD (UAS-salm RNAi;UAS-mito-gfp;mef2)shows fibrillar muscles switched to tubular muscle type and mitochondria (mito-gfp) converted to grid-like networks.g,h,isalm KD; cut KDshows fibrillar fiber type and parallel mitochondrial networks (MitoTracker) in IFMs similar to wildtype.j,k,lcut-OE shows tubular fiber type and grid-like mitochondrial networks (MitoTracker) in IFMs similar tosalmKD (UAS-salm RNAi;UAS-mito-gfp;mef2)(Scale Bars: 5 μm for all).mQuantification of mitochondrial network orientation. Dotted line represents parallel equal to perpendicular (WT IFM,n= 3 animals;salmKD(UAS-salm RNAi;UAS-mito-gfp;mef2)IFM,n= 3 animals;salm KD; cut KDIFM,n= 3 animals; cut-OE, n= 4 animals).nWildtype fibrillar IFM stained for nuclei (DAPI), and salm antibody showing salm expression in the nuclei.osalmKD IFM showing decreased salm expression.pcutKD IFM andqsalm KD; cut KDshowing restored salm expression in the nuclei.rcut-OE showing absence of salm expression in the nuclei (Scale Bars: 5 μm for all).sQuantification ofsalmtranscript levels (WT IFM,n= 5;salmKD (UAS-salm RNAi;UAS-mito-gfp;mef2)IFM,n= 5;cutKD,n= 3;salm KD; cut KDIFM,n=3).tQuantification(qPCR) ofcut,salm, and H15transcript levels. Each point represents value for each dataset. Bars represent mean ± SD. Significance determined asp< 0.05 from one way ANOVA with Tukey’s (*,p≤ 0.05; **,p≤ 0.01; ***,p≤ 0.001; ****,p≤ 0.0001; ns, non-significant). FIB-SEM imaging 2–3 days old flies were dissected on standard fixative solution (2.5% glutaraldehyde, 1% paraformaldehyde, and 0.12 M sodium cacodylate buffer) and processed for FIB-SEM imaging as described previously [31] . Muscles were then transferred to the fresh fixative Eppendorf tube and fixed overnight at 4 °C. Samples were washed in 0.1 M cacodylate buffer for 10 min, three times. Later, fixed tissues were immersed in a solution of 3% KFeCN in 0.2 M cacodylate buffer with 4% OsO 4 on ice for 1 hr. Three washes with distilled water for 10 min each were then performed following incubation in filtered TCH solution for 20 min at room temperature. Three washes with water for 10 min each, then incubated for 30 min in 2% OsO 4 on ice. Incubated samples were washed with distilled water for 10 min, three times each. Tissues were transferred to the freshly made 1% uranyl acetate at 4 °C overnight. Furthermore, samples were washed with distilled water three times for 10 min, then incubated with lead aspartate solution at 60 °C for 30 min. Repeated washing step with warm distilled water and then dehydrated tissues with increasing order of alcohol percentage (20%, 50%, 70%, 90%, 95%, 100%, 100%) at room temperature. Later, samples were transferred to the freshly made 50% Epon resin in alcohol and incubated for 4–5 h at room temperature and then replaced 50% Epon by the 75% Epon incubated overnight at room temperature. Samples were transferred to the freshly prepared 100% Epon resin and incubated for 1 h, repeated the step, and finally transferred to the 100% Epon for 4 h. Tissues were transferred to the stub with as little resin as possible and tissues were incubated for polymerization on the stub for 48 h at 60 °C. FIB-SEM images were acquired using a ZEISS Crossbeam 540 with ZEISS Atlas 5 software (Carl Zeiss Microscopy GmbH, Jena, Germany) and collected using an in-column energy selective backscatter with filtering grid to reject unwanted secondary electrons and backscatter electrons up to a voltage of 1.5 kV at the working distance of 5.01 mm. FIB milling was performed at 30 kV, 2–2.5 nA beam current, and 10 nm thickness. Image stacks within a volume were aligned using Atlas 5 software (Fibics Incorporated, Ontario, Canada) and exported as TIFF files for analysis. Voxel size was set at 10 × 10 × 10 nm. FIB-SEM volumes were segmented in semi-automated fashion using Ilastik [113] machine learning software as described previously [31] . Briefly, FIB-SEM image volumes were binned to 20 nm in ImageJ, saved as 8-bit HDF5 files, and imported into Ilastik. Pixel classification training using all available features was performed for the mitochondria, sarcoplasmic reticulum+t-tubules and all other pixels and exported as 8-bit probability files. The resultant HDF5 files were imported back into ImageJ and binarized using a 50% threshold. The binary structures were filtered using the Remove Outliers plugin in ImageJ using a 3-10 pixel radius and 1.5-2 standard deviations and then rendered in Imaris (Bitplane). Statistics and reproducibility To verify the reproducibility of the original phenotype, we ran a minimum of two independent experiments, which resulted in similar results. Every sample quantified relates to an individual animal, so all samples are biological replicates. Detailed information on the number of samples or animals used for each quantification is shown in the figure legends. Quantitative data were analyzed in Excel 2016 (Microsoft) and statistical tests were performed using Prism 9 (GraphPad). All comparisons of means between Fiber types (IFMs, TDTs, Leg Fiber I, Fiber II, and Fiber III) and between gene knockdown and overexpression groups were performed using one-way analysis of variance with Tukey’s HSD (honestly significant difference) post hoc test. Differences in Cut antibody fluorescence between cut KD and WT were evaluated by comparing the means from each dataset using unpaired t test with Welch’s correction. A p value < 0.05 was used to determine statistical significance. Source data are provided as a Source Data file. Reporting summary Further information on research design is available in the Nature Portfolio Reporting Summary linked to this article.